Self-assembling subnanometer pores with unusual mass-transport properties A long-standing aim in molecular self-assembly is the development of synthetic nanopores capable of mimicking the mass-transport characteristics of biological channels and pores. Here we report a strategy for enforcing the nanotubular assembly of rigid macrocycles in both the solid state and solution based on the interplay of multiple hydrogen-bonding and aromatic π−π stacking interactions. The resultant nanotubes have modifiable surfaces and inner pores of a uniform diameter defined by the constituent macrocycles. The self-assembling hydrophobic nanopores can mediate not only highly selective transmembrane ion transport, unprecedented for a synthetic nanopore, but also highly efficient transmembrane water permeability. These results establish a solid foundation for developing synthetically accessible, robust nanostructured systems with broad applications such as reconstituted mimicry of defined functions solely achieved by biological nanostructures, molecular sensing, and the fabrication of porous materials required for water purification and molecular separations. Developing synthetically accessible constructs with ever increasing functional diversity and complexity is a long-term goal of chemical science [1] . Biological nanotubular complexes, such as the non-selective pore formed by α-hemolysin [2] , and the highly selective channels of ions [3] and water [4] , provide some of the most spectacular examples of supramolecular assemblies with extraordinary structural and functional sophistication. Taking lessons from biological assemblies, the recent integration of molecular design and synthesis with noncovalent forces such as hydrogen-bonding, electrostatic, hydrophobic, π−π and ion–π interactions, along with metal–organic architectures and covalent capture of supramolecular assemblies, has made a significant inroad towards producing various synthetic channels and pores, either from organic building blocks or from cyclic peptides [5] , [6] , [7] , [8] , [9] , [10] , [11] , [12] , [13] . Many of these synthetic molecular and supramolecular structures exhibit interesting mass-transporting properties. Nevertheless, the creation of synthetic channels and pores with structural uniformity and functional selectivity, such as transport of specific ions and molecules, still presents major challenges. In comparison to biological ion channels, most synthetic pores available are hydrophilic with poor ion selectivity, and only a few have demonstrated evidence for water transport [14] , [15] . A conceptually straightforward strategy for constructing synthetic pores involves the stacking of macrocycles, an area that has witnessed impressive progress in recent years [16] , [17] . Of particular interest are molecular-scale (<2 nm) nanopores with fixed sizes, on the basis of which many fascinating properties resulting from confinement within a nanospace, such as selective transport of molecules and ions with significantly enhanced rate, could be realized. The availability of nanopores with these features relies on rigid macrocyclic building blocks that allow convenient synthetic manipulation of their size and function, and carry encoded information that instructs their own stacking and alignment. In addition, the diameters of the resultant nanopores would be defined by their macrocyclic molecular components. Synthetically tuning and modifying the constituent macrocycles allow direct control of the size and surface chemistry of the corresponding nanotubes and their internal pores. This strategy is especially useful for creating nanopores with diameters of 2 nm or less, the most appropriate dimension that exhibits many unusual properties [18] . Molecular-scale nanopores are technically challenging for currently known techniques such as electron-beam lithography (pore size ~5–10 nm) [19] or track-etching (pore size typically ≥10 nm) [20] that are used to fabricate polymer or solid-state films with low surface pore densities. To date, several classes of planar, rigid macrocycles have been reported, including those based on arylene ethynylene backbones [21] , [22] and recently reported ones with aryl amide and hydrazide [23] or Schiff base [24] backbones that can be efficiently prepared. With their persistent shapes unaffected by synthetic modifications, these macrocycles provide an attractive class of building blocks for forming nanotubular assemblies containing internal pores of defined diameters. However, it remains a major challenge to develop practical strategies for stacking shape-persistent macrocycles into columnar assemblies, which requires not only directional, but also positional correlation between the macrocyclic molecules. For example, arylene ethynylene macrocycles have been extensively studied for their aggregation via aromatic stacking [25] . Although tubular assembly is observed with a few structures in the solid state [26] , [27] , the packing of analogous macrocycles, with very small structural differences, varies significantly and in most cases, does not result in a truly tubular arrangement [25] , [28] . Here we describe the creation of organic nanotubes based on the stacking of shape-persistent macrocycles enforced by the cooperative interaction of π−π stacking [29] and hydrogen bonding. In both the solid state and solution, helical nanotubes with modifiable surfaces and a defined, noncollapsible inner pore are obtained. The resultant nanopore, in spite of being hydrophobic, exhibits unusual mass-transporting capabilities including highly selective ion conductance and efficient water transport across lipid membranes. Design of macrocyclic building blocks for nanotubular assemblies The feasibility of a directed stacking strategy is explored based on macrocycles 1a–d , which share a planar, π-conjugated hexa( m -phenylene ethynylene) ( m -PE) core [21] that bears six amide side chains ( Fig. 1a ). Macrocycles 1a and 1b have the same internal cavity but differ in their amide side chains while 1c has the same side chains as those of 1a but has two methyl groups in its internal cavity. Compound 1d , which cannot self-associate via hydrogen bonding, serves as a control. Given the directionality and strength of multiple hydrogen-bonding interactions, macrocycles 1a–c are expected to undergo directional aggregation. To form the maximum number of hydrogen bonds, adjacent macrocycles must stack cofacially, leading to a cylindrical assembly that is encased in sixfold hydrogen-bonded networks. 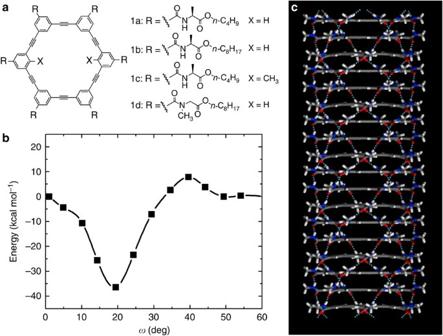Figure 1: Self-assembling macrocycles and their predicted nanotubular structure. (a) Designs of macrocycles1a–cfor assembling into hydrogen-bonded nanotubes, and1dthat is incapable of associating via hydrogen bonding for comparison. (b) The potential energy as a function of the stacking angle (ω) between two stacking macrocyclic units. (c) A snapshot of a helical stack of the macrocycles at the end of the 5 ps QMD simulation. Here all amide side chains are pointing to the same direction. Other assemblies of similar stability are found inSupplementary Fig. S2e. Colour code: O (red), N (blue), C (grey), H (white). Light blue dotted lines refer to hydrogen bonds. Figure 1: Self-assembling macrocycles and their predicted nanotubular structure. ( a ) Designs of macrocycles 1a – c for assembling into hydrogen-bonded nanotubes, and 1d that is incapable of associating via hydrogen bonding for comparison. ( b ) The potential energy as a function of the stacking angle ( ω ) between two stacking macrocyclic units. ( c ) A snapshot of a helical stack of the macrocycles at the end of the 5 ps QMD simulation. Here all amide side chains are pointing to the same direction. Other assemblies of similar stability are found in Supplementary Fig. S2e . Colour code: O (red), N (blue), C (grey), H (white). Light blue dotted lines refer to hydrogen bonds. Full size image Computational studies Ab initio calculations are first performed to evaluate the structure of the assembled complex. The optimal stacking angle is first determined by calculating the potential energy surface of two macrocyclic units, which share the m -PE core and the amide moiety of la and lb , as a function of relative stacking angle, ω . At each given value of ω , the geometry is fully optimized using density-functional theory. As shown in Fig. 1b , the lowest-energy configuration (the global minimum) of this dimer corresponds to a value of 19.5° for ω . In this state, the N-H···O hydrogen bonds between neighbouring macrocycles are perfectly formed, along with an inter-backbone stacking distance of 3.46 Å typical of strong π−π stacking interaction. With this optimal stacking angle determined, an assembly that is infinitely long along the stacking direction is constructed. With three stacked macrocycles per unit cell, this structure is subjected to optimization using a periodic density-functional theory method, which results in a well-defined helical nanotubular structure ( Supplementary Fig. S1 ). The stability of the optimized nanotube is further examined by performing quantum molecular dynamics (QMD) simulations for several picoseconds at 290 K. A snapshot of the assembly at the end of the QMD simulation ( Fig. 1c ), and a Supplementary Video ( Supplementary Movie 1 ) demonstrate that the helical nanotubular structure is indeed stable. It needs to be pointed out that the model shown in Fig. 1c , where all the six amide side chains of the macrocycle point to the same (up or down) direction, is only one of eight possible combinations of the up and down orientations of amide side chains, and all of these assemblies have a similar stability ( Supplementary Fig. S2 ). The same conclusion is also obtained from additional classical molecular dynamics (MD) simulations ( Supplementary Fig. S3 ). Characterization of the nanotubular self-assembly of macrocycles Having established a theoretical basis for nanotubular assembly and stability, macrocycles 1 are synthesized based on Pd-catalysed (Sonagashira) coupling [30] of noncyclical trimeric precursors ( Supplementary Fig. S4 ). X-ray diffraction analysis on a solid sample of 1b , prepared from a solution in chloroform, provides detailed parameters supporting the stacking of the macrocyclic molecules into nanotubes ( Supplementary Fig. S5 ). The diffractogram reveals a dominant peak at 28.08 Å and two other prominent peaks at 16.13 Å and 13.98 Å, with ratios of d -spacings of about 1:1/ :1/2, indicating that there are columns of 1b packed in a hexagonal lattice [31] ( Supplementary Fig. S5b ). The 28.08-Å reflection indicates an intercolumnar distance, or column diameter, of 32.4 Å, which, assuming partially (~8%) collapsed or interdigitated side chains, is consistent with the molecular dimension of 1b . In addition, there is a broad maximum around ~4.2 Å that is typically observed with the columnar phases of discotic liquid crystals [31] . This broad reflection can be identified as the distance between the packed side chains of 1b . Moreover, there is a sharp peak at 3.53 Å, indicative of strong π−π stacking interactions that can be attributed to the interplanar reflection between the flat macrocyclic backbones. Applying Scherrer's equation [32] to this 3.53-Å reflection, an extraordinary long-range ordering of the macrocycles can be inferred within a column, exhibiting a correlation length between 23 nm to 26 nm, corresponding to a nanotube of ~65 to 73 continuously stacked macrocyclic units. Additional structural information of the self-assembling nanotubules formed by 1a and 1b on a solid surface is obtained using atomic force microscopy (AFM) ( Fig. 2 ), scanning electron microscopy (SEM) and transmission electron microscopy (TEM) ( Supplementary Fig. S6 ). These macrocycles readily form very long fibres on solid surfaces as shown by SEM and TEM images. Long and closely packed uniform nanofilaments, each with roughly the same height, are revealed in the AFM images of 1a ( Fig. 2a ) and 1b ( Fig. 2b ). By varying the imaging force systematically and extrapolating the observed heights, a 'zero force' height of 3.2±0.1 nm is obtained ( Supplementary Fig. S7 ). The interfilament distance, a good estimate of the nominal diameter of closely packed nanotubules, is found to be 3.7±0.1 nm. Similar to the assembly of 1a and 1b , the AFM image of 1c also reveals nanotubules ( Fig. 2c ). In contrast, macrocycle 1d , which bears tertiary amide side chains, could not assemble into any regular aggregates ( Supplementary Fig. S8 ). 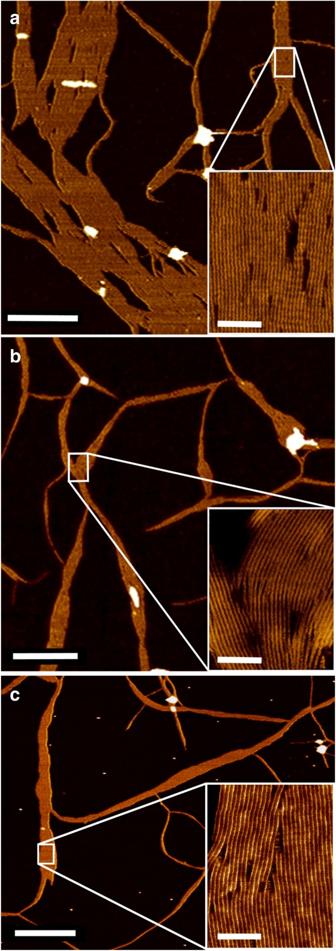Figure 2: Direct observation of self-assembled nanotube structure. Tapping mode AFM images of1a(a),1b(b) and1c(c) assembled in CCl4and deposited on mica. Insets: higher magnification revealed uniform nanofilaments closely packed into quasi-parallel aggregates. In each image, the scale bar for the main image and the inset is 500 nm and 40 nm, respectively. Figure 2: Direct observation of self-assembled nanotube structure. Tapping mode AFM images of 1a ( a ), 1b ( b ) and 1c ( c ) assembled in CCl 4 and deposited on mica. Insets: higher magnification revealed uniform nanofilaments closely packed into quasi-parallel aggregates. In each image, the scale bar for the main image and the inset is 500 nm and 40 nm, respectively. Full size image Having demonstrated the directed stacking of 1a and 1b in the solid state, the solution-phase aggregation of 1b is then probed by ultraviolet and fluorescence spectroscopy ( Supplementary Figs S9 and S10 ). Macrocycle 1b is found to undergo significant aggregation in carbon tetrachloride (CCl 4 ) at micromolar concentrations. In contrast, within the same concentration range, no obvious aggregation of 1b is observed in chloroform, THF, or DMF, solvents with greater polarity compared with CCl 4 . The ultraviolet and fluorescence spectra of 1d , which is incapable of self-association via hydrogen bonding, provide no evidence of aggregation in CCl 4 , or in any of the other solvents ( Supplementary Fig. S9 ). Strong signals around 273 nm, which is the λ max of the absorption spectrum, are evident in the CD spectra of 1b in CCl 4 ( Supplementary Fig. S11 ). The CD spectra of 1b recorded at different temperatures ( Supplementary Fig. S11a ) or concentrations ( Supplementary Fig. S11b ) are similar. Besides, an isodichroic point, consistent with the presence of the same chiral assembly, is present at 282 nm. It is also observed that the concentration-dependent CD spectra of 1b in CCl 4 and those from thin films ( Supplementary Fig. S11d ) are very similar, which correlates the solution-phase assembly of 1b to that in the solid state. In spite of the presence of two methyl groups in its cavity, the CD spectra of 1c ( Supplementary Fig. S11c ) have the same overall features as those of 1b . Transmembrane ion transport through self-assembled nanopores With their hydrophobic side chains, it is expected that macrocycles 1a–c could partition into the hydrophobic core of lipid bilayers, and self-assemble into transmembrane nanopores. When a solution of large unilamellar vesicles (LUVs) enclosing a pH-sensitive dye, HPTS, is subjected to an extravesicular pulse of HCl, followed by addition of 1a , a significant, concentration-dependent, and faster decrease of fluorescence emission from the entrapped HPTS was indeed observed ( Fig. 3a ) [33] . The addition of Triton X-100, a nonionic surfactant known to completely rupture the LUVs, results in a nearly instantaneous, complete reduction of the fluorescence emission ( Fig. 3a ). In contrast to 1a , macrocycle 1c , which bears the same side chains as 1a but has two methyl groups in its cavity, does not result in any detectable change on the rate of fluorescence change ( Fig. 3a ). 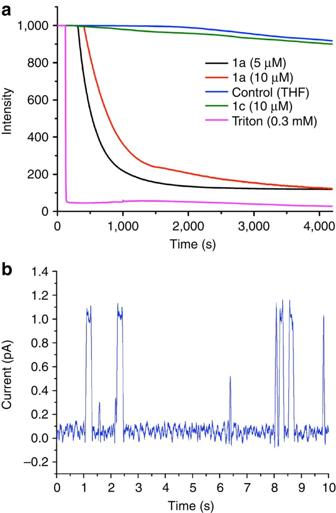Figure 3: Enhanced membrane permeability mediated by 1a. (a) Time-dependent changes in fluorescence intensity of 8-hydroxypyrene-1, 3, 6-trisulfonate (HPTS, 0.1 mM) encapsulated inside large unilamellar vesicles (LUVs) of 1-palmitoyl-2-oleoyl-sn-glycero-3-phosphocholine and phosphatidyl serine (4:1 mass%). Solutions of LUVs (HEPES, pH 7.2) with1aor1c(added from 1-mM stock solutions in THF), and without added1aor1cwere first incubated for 1 min, each of which was then acidified with an acid pulse (40 μL of 2M HCl) followed by monitoring the change of emission intensities over time. Total LUV disruption is achieved with 0.3 mM Triton X-100. (b) A 10-s single channel recording with1a(20 μM) at 200 mV in HCl (1 mM) across a planar lipid bilayer. Figure 3: Enhanced membrane permeability mediated by 1a. ( a ) Time-dependent changes in fluorescence intensity of 8-hydroxypyrene-1, 3, 6-trisulfonate (HPTS, 0.1 mM) encapsulated inside large unilamellar vesicles (LUVs) of 1-palmitoyl-2-oleoyl-sn-glycero-3-phosphocholine and phosphatidyl serine (4:1 mass%). Solutions of LUVs (HEPES, pH 7.2) with 1a or 1c (added from 1-mM stock solutions in THF), and without added 1a or 1c were first incubated for 1 min, each of which was then acidified with an acid pulse (40 μL of 2M HCl) followed by monitoring the change of emission intensities over time. Total LUV disruption is achieved with 0.3 mM Triton X-100. ( b ) A 10-s single channel recording with 1a (20 μM) at 200 mV in HCl (1 mM) across a planar lipid bilayer. Full size image To delineate the nature of the observed increase in proton influx, single-channel electrophysiology is performed with planar lipid bilayers to which 1a is added through the aqueous phase [34] . Consistent with the formation of individual ion channels, macrocycle 1a indeed can form well-defined single conductance steps in 1 mM HCl ( Fig. 3b ). By measuring the reversal potential under asymmetric salt solutions, this 1a channel is found to have a high proton (H + ) selectivity, exhibiting a P H +/P Cl − ratio of greater than 3,000 ( Supplementary Fig. S12 ). With such a marked selectivity for protons over chloride, whether other monovalent cations would also conduct through the 1a channel is further investigated. In concentrated KCl (4 M) solution, there is indeed a small, but measurable and well-defined single-channel current ( Fig. 4a ) with a mean conductance of ~5.8 pS. Combining the results for proton conductance with those for potassium, a permeability ratio, P H+ /P K+ , of ~2,000 is inferred. At similar concentrations of either NaCl or LiCl, no transmembrane current is detected ( Supplementary Fig. S13 ), illustrating a striking selectivity of these channels. 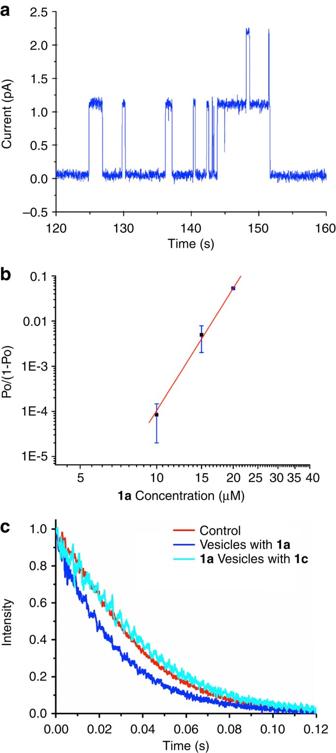Figure 4: Ion- and water-transporting properties of self-assembled nanotubes. (a) A 160-s trace of single-channel recording with1a(10 μM) at 200 mV in KCl (4.0 M, pH 6.0). (b) Open probability dependence of1aon concentration. The red line is fitted to Hill equation: log(PO/(1−PO))=nlog([1a])−log(K). The results aren=9±3, and EC50=30 μM (21). From low-to-high concentration, the standard deviations are 6×10−5, 3×10−3, and 0.32×10−2(Supplementary Table S1). (c) Water permeability measured with CF-containing liposomes in the presence (blue) and absence (red) of1aand with1c(cyan). The lipid to1aor1cratio is 50. LUVs were abruptly exposed to a high extra-vesicular osmolality of 435 mM NaCl in a stopped-flow instrument, with a final osmolarity ratio of 3. The LUVs with1ashowed clearly a faster decay of fluorescence in comparison to those without or with1c. Figure 4: Ion- and water-transporting properties of self-assembled nanotubes. ( a ) A 160-s trace of single-channel recording with 1a (10 μM) at 200 mV in KCl (4.0 M, pH 6.0). ( b ) Open probability dependence of 1a on concentration. The red line is fitted to Hill equation: log(P O /(1−P O ))=nlog([ 1a ])−log(K). The results are n =9±3, and EC50=30 μM (21). From low-to-high concentration, the standard deviations are 6×10 −5 , 3×10 −3 , and 0.32×10 −2 ( Supplementary Table S1 ). ( c ) Water permeability measured with CF-containing liposomes in the presence (blue) and absence (red) of 1a and with 1c (cyan). The lipid to 1a or 1c ratio is 50. LUVs were abruptly exposed to a high extra-vesicular osmolality of 435 mM NaCl in a stopped-flow instrument, with a final osmolarity ratio of 3. The LUVs with 1a showed clearly a faster decay of fluorescence in comparison to those without or with 1c . Full size image An analysis [35] of the open/close probability under different concentrations of 1a in 4 M KCl leads to a fitted Hill coefficient ( Fig. 4b ) of 9±3, consistent with the self-assembly of at least nine molecules of 1a to form a functional transmembrane channel. This stoichiometry is also confirmed by MD simulations, which indicate that the most probable stoichiometry for the transmembrane channel of 1a in a lipid bilayer is 10 ( Supplementary Fig. S14 ). Direct measurement of transmembrane water transport We noted recent studies on carbon nanotubes showing that water can spontaneously fill small hydrophobic nanopores [36] , [37] , especially those with small pore diameters [36] , [37] , [38] , [39] , [40] , [41] , [42] , leading to enhanced mass flow or resonance [40] , [43] . The observed ion conductance of the hydrophobic channel formed by 1a implies that this sub-nm pore may also be filled with water molecules. To directly validate this possibility, stopped-flow kinetic measurements on 1a -containing LUVs loaded with carboxyfluorescein (CF), a technique that monitors the volume change of liposomes and was previously used to measure the water channel activity of aquaporin 1 (AQP1, CHIP-28) [44] , are conducted. By increasing the osmolarity outside the LUVs [45] , the net flow of water molecules out of the vesicles should increase, leading to a reduced volume of liposomes and increased self-quenching of the trapped CF. The rate of fluorescence reduction is thus a reflection of the water permeability of the constituting membrane. As shown in Fig. 4d , LUVs with incorporated 1a exhibit a noticeably faster decay of fluorescence (blue) than those without 1a (red) or with 1c (cyan), and the rate of this decay is directly dependent on the 1a -to-lipid ratio ( Supplementary Fig. S15 ). The osmotic water permeability coefficient, P f , is 0.0051 cm s −1 for LUVs with a diameter of ~100 nm prepared from a lipid/ 1a molar ratio of 50, in comparison to a value of P f of 0.0044 cm s −1 obtained for the same sized LUVs without 1a . Assuming that the channels formed in the LUV's have a similar kinetic behaviour as found by single-channel recordings, with each channel requiring about 10 monomers and an open probability of ~5%, the estimated water permeability ( P f ) of a single 1a channel is 2.6 (±0.4)×10 −14 cm 3 s −1 when open, about 22% of that of AQP1/CHIP-28 (11.7×10 −14 cm 3 s −1 ) [44] . The tubular assembly of macrocycles 1 revealed by computational studies satisfies both the optimal distances of side-chain hydrogen bonding and the backbone π−π stacking interactions ( Supplementary Fig. S2 ), which results in a helical stack of macrocycles encased in sixfold hydrogen-bonded networks. Such a self-assembling nanotube has a defined, internal van der Waals diameter of 6.4 Å. Similar to the hydrophobic pores of carbon nanotubes, the internal lumen of the self-assembling nanotubes, described here, is also hydrophobic and has a fixed diameter, because of the persistent shape of its macrocyclic components. In contrast to the smooth, π-electron-rich interior surface of carbon nanotubes, the interior surface of this self-assembling hydrophobic pore is decorated with numerous inward-pointing aromatic hydrogen atoms and is expected to have different properties. Consistent with the computational prediction, the efficient formation of very long fibres on solid surfaces indicates the high propensity of macrocycles 1a and 1b for anisotropic assembly. This observation confirms the expected high directionality of the self-assembly of the designed macrocycles, which is typical of intermolecular association mediated by multiple hydrogen-bonding interactions. The interfilament distance (3.7 nm) measured for 1a on solid surface by AFM and the intercolumnar distance (3.2 nm), revealed by X-ray diffraction on the bulk sample of 1b , are in good agreement with the estimated diameter of 1a (~3.8 nm assuming fully extended side chains) and similarly with that of 1b , suggesting that these macrocycles indeed stack on top of one another and align co-axially. The AFM image of 1c , which differs from 1a by having two methyl groups in its cavity, shows that methylation of the inner cavity does not have any observable effect on the self-assembly of the macrocycle and thus the formation of the corresponding nanotubes. In contrast, the inability of macrocycle 1e , which is incapable of undergoing hydrogen bond-mediated self-assembly, to generate analogous fibrous and tubular structures illustrates the critical importance of hydrogen bonding in forming the self-assembling nanotubes observed for 1a–c . For 1b , the lack of aggregation revealed by CD, in solvents of enhanced polarity, provides additional support for the significance of hydrogen bonds in self-assembly. The strong CD signals exhibited by 1b in CCl 4 indicate the presence of an assembly with a chirality that is biased by the transfer of chirality from the ultraviolet-silent side chains to the m -PE macrocyclic backbone. Chiral arrangement of the m -PE backbone corroborates the helical stack predicted by computations. The similar shape of the CD spectra of 1b at different temperatures ( Supplementary Fig. S11a ) or concentrations ( Supplementary Fig. S11b ), and the presence of the isodichroic point at 282 nm, suggest that the aggregated structure adopts the same chirality under all of these conditions. Finally, the similarity in the CD spectra of 1b , obtained under solid-state and solution-phase conditions, ( Supplementary Fig. S11 ) provides additional evidence that the helical nanotubular assemblies revealed in the solid state also persists in solution. In CCl 4 , macrocycle 1c gives strong CD signals that resemble the features observed for those of 1b . Such an observation, along with the similar AFM images of 1a–c , indicates that modifying the internal cavity with methyl groups does not disturb the formation of the nanotubular assemblies in either solid state or in solution, suggesting a possibility of using other modifications to achieve different functions in these nanopores. The robustness of this nanotubular assembly is likely the key reason for its ability to readily form transmembrane channels. The observed fluorescence quenching of HPTS entrapped in LUVs indicates that 1a can indeed partition into lipid bilayers and alter membrane permeability. The observed leveling off of the fluorescence emission at later times, after adding 1a ( Fig. 3a ), can be explained by the reversal potential [3] that forms as a consequence of a greater proton permeability than that of chloride, which hinders further proton influx (see Supplementary Methods ) [33] . Given that 1c differs from 1a only in the two methyl groups in its cavity, the inability of 1c to effect fluorescence quenching suggests that the presence of the methyl groups in the cavity of 1c serves to hinder proton influx, which in turn indicates that the enhanced rate of proton influx mediated by 1a is due to transport through the interior of the macrocycles, that is, through the lumen of the transmembrane nanopores formed by 1a . That the self-assembling nanopores of 1a serve as transmembrane channels is directly demonstrated by the detection of single-channel conductance ( Figs 3b and 4a ) and the remarkable selectivity of the corresponding ion-transporting activity. The measured H + /Cl − selectivity (~3,000) is much higher than that of natural proton channels, such as the influenza virus M2 protein (P H +/P Cl −=19.7) [46] , even though the mechanism of selectivity with this artificial channel is apparently different from that of a protein channel. The observed H + /K + selectivity (~2,000), although not as high as the M2 channel (10 7 ), is still significant when compared with other known synthetic channels [47] . The fact that the self-assembling nanopore formed by 1a is both hydrophobic and ion selective reinforces the notion [48] , [49] that the transport of ions within a small (sub-nm to 2 nm) nanochannel can be highly sensitive to the precise nature of the specific ions. For instance, compared with K + conductance that requires physical diffusion, proton transport could be much more efficient based on an orientational hydrogen-bonding defect mechanism [50] , [51] . Here the observed K + /Na + selectivity can be understood based on conclusions from previous MD simulations [48] , [49] , which demonstrates that the free-energy costs of constraining hydrated K + within a sub-nm pore are notably less than those of hydrated Na + . The stoichiometry of the 1a channel determined experimentally ( Fig. 4b ) or from MD analysis ( Supplementary Fig. S14 ) corresponds to a nanopore consisting of 9 to 10 stacked macrocyclic molecules. Given that the typical π−π stacking distance is about 3.6 Å, the length of a transmembrane stack of 1a matches closely the thickness (3 to 4 nm) of the hydrophobic core of a lipid bilayer, suggesting that the observed tranmembrane ion transport is indeed mediated by the self-assembling nanopore of 1a . Such assembly apparently requires a proper balance of hydrogen bonding, π−π interaction and side-chain interaction with the hydrophobic core of the lipid bilayer. Yet, even more remarkable than the observed ion conductance and especially the high selectivity in ion translocation, the hydrophobic 1a nanopore demonstrates an impressive efficiency of water transport that is about 22% of that of aquaporin 1. Although the structure of 1a nanopore is significantly different from that of a carbon nanotube, the observed efficient water transport suggests that efficiency in water transport may be a general phenomenon that is associated with geometrically constrained hydrophobic nanospace. In other words, small, hydrophobic pores may all have high water flux. Elucidating the mechanism for the observed water conductance by these readily tunable self-assembling nanopores could lead to new insights into mass transport under nanoconfinement. The observation that 1c ( Fig. 3c ), with a cavity containing two methyl groups ( Fig. 1a ), failed to produce any increased water permeability further supports the conclusion that the lumen of the self-assembled nanopores is the conduit for transport. This work demonstrates that the interplay of multiple hydrogen bonding and π−π stacking interactions is a reliable, general strategy for controlling the alignment of shape-persistent macrocycles into well-defined nanotubes. The versatile transporting capabilities of the well-defined hydrophobic pore of the 1a channel demonstrate the great potential of the strategy, described here, in controlling size and creating functions, such as high selectivity and high flux, properties that are still elusive for other synthetic nanopores known thus far. The ready synthetic availability and modifiability of many shape-persistent macrocycles offer molecular-level controllability and tunability on the self-assembling nanotubes, which should lead to a variety of novel organic nanotubes with inner pores of defined widths and tunable properties. These discrete nanoporous structures, which are beyond the reach of current fabrication methods, may lead to the discovery of additional unique and unusual functions expected of the nanometer and subnanometer size regime and thus provide new opportunities for fields such as chemical and biological separation, sensing, and catalysis [52] . Materials and instrumentation Chemicals were purchased from commercial sources and used as received. Reactions requiring an inert gas were all under nitrogen. The 1 H NMR spectra were recorded at 400 or 500 MHz and 13 C NMR spectra were measured at 100 or 125 MHz on a Bruker AV400 or AV500 spectrometer at ambient temperature. Ab initio computation and QMD simulation were carried out on Firefly Supercomputer (University of Nebraska Holland Computing Center) using a density functional theory method, implemented in the CP2K 2.2 software package 53 . Specifically, for the QMD simulation, the supercell of the periodic system consist of three stacked macrocycles in view of the optimal stacking angle ω being ~20°. The isothermal–isobaric (NPT) ensemble is used for the QMD simulation with flexible simulation cell, and the external pressure is 1 atm. The temperature of the system is controlled at 290 K. The simulation time is 5.0 ps with the time step of 1.0 fs. Classical molecular dynamics simulations of 1a nanotube in vacuum, water and chloroform were performed using GROMACS 3.3.3 and NAMD 2.7, respectively. X-ray diffraction was recorded at the 2-ID-D beamline of the Advanced Photon Source at Argonne National Laboratory using 10.1 keV radiation (λ=1.2275 Å) on a Newport 6-circle (Kappa) diffractometer. Without gold coating, TEM images were obtained using a Hitachi S-4800 scanning electron microscope, with an acceleration voltage of 3 kV. TEM measurements were imaged on holey carbon films using a Tecnai G2 F20 U-TWIN transmission electron microscope, operated at 120 kV or 200 kV. AFM images were recorded using a Nanoscope 3D multimode SPM (Veeco Instruments, Santa Barbara, CA, USA) in air with the tapping mode, using RTESP probes (40 N m −1 , 300 kHz, Veeco Probes, Camarillo, CA, USA). Synthesis of macrocycles 1 The synthesis of and isolation of macrocycle 1a , based on Pd-catalysed coupling of the corresponding di-iodo- and di-ethynyl-terminated PE trimers, is given as an example. Under nitrogen protection, Pd 2 (dba) 3 (0.03 g, 0.033 mmol), CuI (0.02 g, 0.076 mmol) and PPh 3 (0.09 g, 0.47 mmol) were added to a 250 ml round-bottomed flask with two necks, heated to reflux, followed by addition of DMF (120 ml) and NEt 3 (30 ml) via syringe, then the solution of the di-iodo-terminated PE trimer (0.05 g, 0.048 mmol) and di-ethynyl-terminated PE trimer (0.038 g, 0.048 mmol), in 10 ml DMF, was slowly injected by a syringe pump into the flask within 48 h. The reaction mixture was refluxed for another 12 h and was then concentrated in vacuo , leaving a residue that was purified by column chromatography (silica gel, CH 2 Cl 2 /THF=25:1) to give the desired product (0.01 g, 12.6%) as a white solid. 1 H NMR (400 MHz, DMF) δ 9.15 (d, J =6.7 Hz, 6H), 8.22 (s, 12H), 8.07 (s, 6H), 4.62 (m, 6H), 4.12 (m, 12H), 1.62 (m, 12H), 1.56 (m, 18H), 1.38 (m, 12H), 0.90 (t, J =7.4 Hz, 18H); 13 C NMR (100 MHz, DMF) δ 172.9, 165.1, 137.4, 135.6, 130.9, 123.5, 89.3, 64.6, 49.4, 30.8, 19.1, 16.7, 13.4; MS (MALDI-TOF): 1,650.1 [M+Na] + . Proton flux across lipid bilayers Liposomes (LUVs) were prepared from phospholipids POPC (1-palmitoyl-2-oleoyl-sn-glycero-3-phosphocholine)/PS ( L -α-phosphatidylserine) (from Avanti Polar Lipids, Alabaster, AL, USA) in an 80/20 (w/w) ratio dissolved in chloroform. The solvent was then evaporated under reduced pressure using a stream of nitrogen for at least 2 h, after which the lipid film was placed in a buffer (100 mM HEPES, 145 mM NaCl, pH 7.2; final concentration of lipids=50 mg ml −1 ) containing the pH-sensitive dye 8-hydroxypyrene-1, 3, 6-trisulfonic acid (HPTS, 0.1 mM). The solution was hydrated in a water bath for at least 1 h followed by five freeze-thaw cycles, with each cycle consisting of alternate freezing (10 min) and heating (10 min) with a quick vortex in between the two extremes. On completing the last cycle, the large multilamellar vesicles were equilibrated for 15 min before their extrusion through a 0.1-μm polycarbonate membrane (Avanti) to produce a homogeneous solution of large unilamellar vesicles (LUVs). LUVs were then separated from the extravesicular fluorescent dye by gel filtration using a 10DG desalting column (Bio-Rad Laboratories) pre-equilibrated with the HEPES buffer. Change of membrane permeability mediated by compounds 1a and 1b was then studied by pulsing the solutions of the prepared LUVs at neutral pH with an aliquot (40 μl) of a HCl (2.0 M) solution. In the presence of transmembrane pores, the fluorescence intensity of HPTS is quenched by the influx of protons through the pores. Single-channel conductance across lipid bilayers Details of preparing planar lipid bilayers is found else where [54] , [55] . Briefly, DPhPC (Avanti) lipid, dissolved at 10 mg ml −1 in chloroform, was dried under a stream of nitrogen for a few minutes. The lipid was then dispersed in decane at 40 mg ml −1 . This mixture was used to pre-coat a 200-μm aperture on the outer side of a Delrin cup (Warner Instruments, Hamden, CT) on which a planar lipid bilayer membrane was formed at room temperature within a chamber having 1 ml saline solution (HCl, KCl, NaCl or LiCl) on both sides. Formation of the membrane was monitored by microscopy and membrane capacitance. The test compound ( 1a or 1b ) in THF (1 mM) was added to both sides of the chamber to a final concentration of 5~20 μM. A holding potential of +200 mV was applied and the channel current was recorded. Channel activity was measured with respect to the trans (ground) side. Ag/AgCl electrodes were used to apply bias voltages and to record currents across the membrane [34] . After observation of the channel activity, the voltages across the lipid bilayer were varied between −200 mV to +200 mV to determine the current (I)–voltage (V) relationship. A Warner Instruments planar lipid bilayer workstation was used for all experiments. Data were amplified (BC-525D Bilayer Amplifier; Warner), digitized (NI PCI6110; National Instruments, Austin, Texas, USA), filtered (LPF-8; Warner) and stored on a PC using the Signal Express (version 2.5; National Instruments). Data analysis was performed using the Origin 7.5 and home-made Matlab program (version 2007Ra) [34] . After data acquisition, the raw current data is low passed before further processing. The data was sampled at 5 kHz and filtered by 1 kHz. Water transport Stopped-flow measurements were performed with a stopped-flow fluorometer (SX-20, Applied Photophysics, Leatherhead, UK) with a measured dead time of 0.5 ms at 12 °C. The excitation wavelength was set at 493 nm using a 150-W mercury–xenon arc lamp and monochromator, the emission wavelength was (515–555 nm) using a band-pass filter. P f (coefficient of osmotic water permeability) was measured by exposing macrocycle 1a - or 1c -containing liposomes or control liposomes to an osmotic gradient by rapid mixing with an equal volume of another solution (100 mM HEPES, 725 mM NaCl, pH 7.2). The P f was determined by the method described in Zeidel et al . [44] , with the water permeability equation: where V ( t ) is the relative intra-vesicular volume as a function of time, P f is the osmotic water permeability coefficient, SAV is the vesicle surface area to volume ratio, MVW is the molar volume of water (18 cm 3 mol −1 ), and C in , and C out are the initial concentrations of total solute inside and outside the vesicle, respectively. Previous studies have established that, within a reasonable range, the volume change is linearly proportional to the decrease in fluorescence, owing to the increased fluorophore concentration during water efflux. The osmotic water permeability of each open channel, p f , can then be estimated from the P f as follows: where P open is the channel open probability; P f channel is the coefficient of osmotic water permeability of liposomes with 1a channels; P f control is the coefficient of osmotic water permeability of liposomes without 1a channels; N channel is the number of channels in the liposome per unit area. How to cite this article: Zhou, X. et al . Self-assembling subnanometer pores with unusual mass-transport properties. Nat. Commun. 3:949 doi: 10.1038/ncomms1949 (2012).